Generation of ultra-short hydrogen atom pulses by bunch-compression photolysis Ultra-short light pulses enable many time-resolved studies in chemistry, especially when used in pump-probe experiments. However, most chemical events are not initiated by light, but rather by collisions. Time-resolved collisional experiments require ultra-short pulses of atoms and molecules—sadly, methods for producing such pulses are so far unknown. Here we introduce bunch-compression photolysis, an approach to forming ultra-short and highly intense pulses of neutral atoms. We demonstrate H-atom pulses of 1.2±0.3 ns duration, far shorter than any previously reported. Owing to its extraordinarily simple physical principles, we can accurately model the method—the model shows H-atom pulses as short as 110-ps are achievable. Importantly, due to the bunch-compression, large (mm 3 ) photolysis volumes are possible, a key advantage for pulse intensity. This technique overcomes the most challenging barrier to a new class of experiments on time-resolved collisions involving atoms and molecules. Short intense pulses of neutral atoms and molecules have found great utility in many important fields of science, including carbon-cluster spectroscopy [1] , production of ultra-cold molecules [2] , observations of vortices in superfluid droplets [3] as well as investigations of chemical transition states [4] to name just a few. Generally produced by mechanically actuated choppers or valves, pulse durations are limited to a few μs. Just as ultra-short light and electron pulses have become central tools for a wide variety of dynamical studies in physics, chemistry and biology [5] , [6] , [7] , [8] , [9] , [10] , [11] , non-mechanical approaches to produce much shorter pulses of neutral atoms and molecules offer fascinating new experimental possibilities. Timing experiments of all kinds initiated by bimolecular collisions become possible, for example, direct lifetime measurements of bimolecular collision complexes (the lifetimes of collision complexes can be indirectly inferred from scattering angular distributions. See for example, ref. 12 ), time-resolved studies of surface adsorbate equilibration [13] as well as real-time kinetics of thermal desorption from terraces and steps [14] , [15] . Synchronized scattering of ultra-short matter pulses from photo-excited surfaces is another opportunity. Surfaces with novel electronic properties are of particular interest as they can exhibit electronically nonadiabatic interactions with atoms and molecules [16] , [17] , [18] , [19] , due to failure of the Born-Oppenheimer approximation. In contrast to light, producing short neutral matter pulses is fraught with problems. Light is fast—hence, uncertainties in distances between the place where the light pulse is produced and where it is used result in only small timing differences. By contrast, neutral atoms and molecules typically travel at speeds 10 −5 that of light. This suggests we must produce and use neutral matter pulses within extremely small volumes to achieve ultra-short durations. Even more daunting, in non-dispersive media, light travels at a single speed; while neutral matter exhibits speed distributions, often very broad ones. Hence, light pulses once formed stay together, whereas neutral matter pulses spread as they travel in direct proportion to the width of their speed distributions. These problems are illustrated by hydrogen iodide (HI) photolysis using a 20-ns laser light pulse, which produced H-atom pulses at a distance of 15 mm (ref. 20 ). Here, a narrow bandwidth ultraviolet laser ensured the H-atom speed was high—10 km s −1 —and its speed distribution narrow. Despite this, the size of the laser-beam’s focus—1 mm 3 —meant the H-atom pulse could not be shorter than 100 ns (ref. 20 ) due to the spread in flight distances experienced by the ensemble of atomic photoproducts. With smaller laser foci and shorter laser pulses, one might imagine producing shorter H-atom pulses. However, tight focusing reduces the photolysis volume with drastic consequences for H-atom pulse intensity. Moreover, short laser pulses possess large frequency spreads, broadening the speed distribution of the atomic photoproducts. In this work, we demonstrate short pulses of hydrogen atoms produced by short pulse laser photolysis from an extended volume. A position-dependent excitation frequency is employed for photolysis of HI, ensuring faster H-atoms travel farther to the target. The extended photoproduct-bunch compresses in flight, producing an extraordinarily short atomic pulse several cm from the photolysis volume. This approach allows the use of short light pulses and avoids the need for tight focusing. 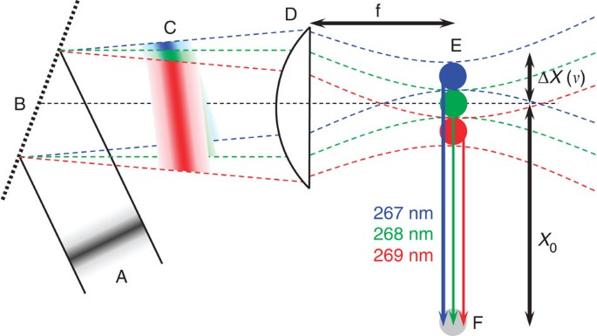Figure 1: Schematic drawing of the working principle of bunch-compression photolysis. The input laser beam (A) is dispersed on a grating (B). The diverging pulse (C) is focused with lens (D) with focal length, f. The single frequency components are focused onto spots with a spatial detuning, ΔX(v), relative to the central frequency. This is depicted in a schematic manner for three selected wavelengths. Owing to the continuous frequency shift, these spots are not separated and yield a focal line (E). The H-atoms are generated by photodissociation at different laser frequencies and emerge with different speeds, such that the initial H-atom photo-product bunch is compressed at spot (F). Demonstrating bunch-compression photolysis Figure 1 shows a schematic of the experiment used to demonstrate the principles of bunch-compression photolysis. A 268-nm Fourier-transform (FT)-limited Gaussian 100-fs laser pulse (A) is dispersed on grating (B), which due to the laser pulse’s frequency spread results in a chirped diverging beam (C) that is then focused with lens (D). The individual frequency components are focused onto spots along a 1.5 mm line focus (E). Higher frequencies are focused further from bunch-compression point (F) than lower ones. As photolysis at higher laser frequency produces faster H-atoms, the bunch of H-atoms generated by photodissociation compresses as it flies towards the bunch-compression point (F). With the proper spatial distribution of frequencies, the H-atoms will arrive nearly simultaneously at (F). Varying the angle of incidence of the laser beam on the grating (B) tunes the spatial frequency distribution allowing us to optimize the bunch-compression. Figure 1: Schematic drawing of the working principle of bunch-compression photolysis. The input laser beam (A) is dispersed on a grating (B). The diverging pulse (C) is focused with lens (D) with focal length, f. The single frequency components are focused onto spots with a spatial detuning, Δ X ( v ), relative to the central frequency. This is depicted in a schematic manner for three selected wavelengths. Owing to the continuous frequency shift, these spots are not separated and yield a focal line (E). The H-atoms are generated by photodissociation at different laser frequencies and emerge with different speeds, such that the initial H-atom photo-product bunch is compressed at spot (F). 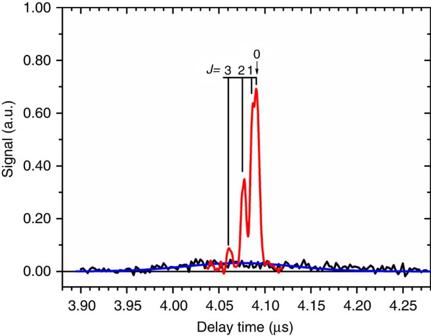Figure 2: Ultra-short H-atom pulse train produced by bunch-compression photolysis. H-atom pulses measured at a distanceX0=44.6 mm from the photolysis region generated with (red) and without (black) bunch-compression. The H-atom pulse generated by bunch-compression photolysis shows several peaks, which originate from different rotational states of the parent HI molecule indicated by the rotational quantum number,J. Both signals were obtained under otherwise identical experimental conditions and the curves are scaled to photolysis laser pulse energy. The blue curve is the pulse expected due to the photon energy spread of the laser pulse. Full size image Figure 2 demonstrates the effectiveness of bunch-compression photolysis. The black curve shows the H-atom pulse produced by a tightly focused 100-fs laser pulse, conventional photolysis. Owing to the photon energy spread of the laser pulse and the resulting velocity spread of the H-atom photoproducts, the H-atom pulse has broadened to 135 ns (FWHM) during its flight to the probe volume, fully six orders of magnitude longer than the photolysis laser pulse. The red curve shows the results of bunch-compression photolysis using the set-up shown in Fig. 1 . The pulse duration is reduced so markedly that a pulse train is now seen, resulting from the individual rotational states of HI that are present in the molecular beam. Note that HI rotational energy appears as H-atom kinetic energy; each pulse in the train has a slightly different speed. The pulse arising from a single HI rotational level is two orders of magnitude shorter than that produced with conventional photolysis. Figure 2: Ultra-short H-atom pulse train produced by bunch-compression photolysis. H-atom pulses measured at a distance X 0 =44.6 mm from the photolysis region generated with (red) and without (black) bunch-compression. The H-atom pulse generated by bunch-compression photolysis shows several peaks, which originate from different rotational states of the parent HI molecule indicated by the rotational quantum number, J . Both signals were obtained under otherwise identical experimental conditions and the curves are scaled to photolysis laser pulse energy. The blue curve is the pulse expected due to the photon energy spread of the laser pulse. Full size image The peak intensity of the beam produced by bunch-compression photolysis is 20 times higher than that produced by conventional photolysis. In making this comparison, we normalized the signals to the photolysis laser pulse energy. At the laser energies used for these experiments, conventional photolysis nearly saturates HI dissociation and produces substantial multiphoton ionization. In contrast, the bunch-compression photolysis is about 20 times below saturation and multiphoton processes are unimportant. The markedly larger instantaneous H-atom pulse intensity seen in Fig. 2 for bunch-compression photolysis could be increased at least another order of magnitude by using higher pulse energies. Modelling bunch-compression photolysis Many factors contribute to the shape and intensity of the pulses displayed in Fig. 2 . The key factors controlling pulse duration are explained in Supplementary Note 1 . The temporal and spatial profiles of the photolysis and detection laser pulse, the variation of photolysis pulse frequency along the line (E) in Fig. 1 , and the variation of photolysis and detection probability with the intensities of the laser pulses are all important. To understand this more fully, we performed a numerical simulation of the signal considering all these factors. The numerical model is described in detail in Supplementary Note 2 . First, we employ a ‘short photolysis-pulse approximation’ (see Supplementary Note 3 ). We imagine an instantaneous photolysis pulse with a position-dependent frequency that illuminates the HI molecular beam along the line (E) of Fig. 1 . The model calculates the position of the photolysis volume and corresponding H-atom velocity at a given frequency within the bandwidth of the photolysis laser. The model then performs a Monte-Carlo integration sampling trajectories between points in the photolysis and detection volumes. The weight of each trajectory’s contribution is computed using measured intensity distributions of laser beams together with the measured intensity dependencies of the photolysis and detection steps. This is then repeated for every frequency within the bandwidth of the photolysis laser and finally for each rotational state of HI in the molecular beam. 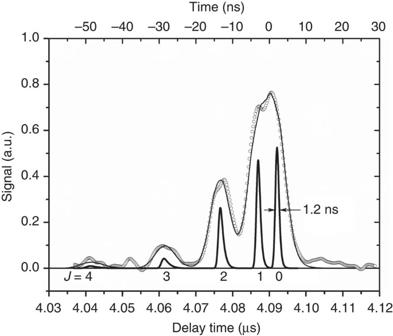Figure 3: Detailed view of the H-atom pulse train obtained with bunch-compression photolysis. The open circles show the observed H-atom pulse train obtained by scanning the delay between the two laser pulses used for photolysis and detection. H-atoms originate from HI, which populates several rotational states in the molecular beam. The thin black line shows the numerical simulation of the observed H-atom signal as detected by sixth order non-resonant ionization from a 100-fs Ti:sapphire laser pulse at 800 nm. The effective detection length is 60 μm. The thick solid line is the prediction of the numerical simulation for a realistic pump-probe experiment where the H-atom pulse collides with a flat surface placed at the bunch-compression position. Figure 3 shows the results of the numerical model (thin solid line) alongside the experimentally observed H-atom pulse train (open circles). We emphasize that the model has no adjustable parameters other than the HI rotational state populations, which determine the amplitude of each pulse in the train. The excellent agreement between model and observation gives us confidence to employ the model to analyse bunch-compression photolysis in more detail. Figure 3: Detailed view of the H-atom pulse train obtained with bunch-compression photolysis. The open circles show the observed H-atom pulse train obtained by scanning the delay between the two laser pulses used for photolysis and detection. H-atoms originate from HI, which populates several rotational states in the molecular beam. The thin black line shows the numerical simulation of the observed H-atom signal as detected by sixth order non-resonant ionization from a 100-fs Ti:sapphire laser pulse at 800 nm. The effective detection length is 60 μm. The thick solid line is the prediction of the numerical simulation for a realistic pump-probe experiment where the H-atom pulse collides with a flat surface placed at the bunch-compression position. Full size image We first note that the observed pulse width, which can be seen clearly in the fully resolved J =2 member of the pulse train, is dominated by the time resolution of our detection scheme, that is, by the effective detection size of the probe laser pulse. The model indicates that the H-atom pulses produced here are substantially shorter. We used our numerical model to simulate the H-atom pulse train under conditions that might be used in an actual pump-probe experiment where H-atom pulses collide at a surface initiating an event that is then followed by a delayed laser pulse. Here, the H-atom pulse is envisioned to collide with a 1 × 1 mm 2 flat surface placed at the bunch-compression distance. The resulting arrival time spread of the H-atoms colliding at the surface is shown as a thick solid line in Fig. 3 . The bunch-compression is best for the J =0 state and slightly degraded for higher rotational states, which travel at different speeds and hence exhibit slightly different bunch-compression distances. The FWHM of the J =0 member of the pulse train is 1.2 ns and represents the actual duration of the shortest H–atom pulses produced in this work. The uncertainty in the pulse duration, ±0.3 ns, results from experimental error in the determination of the size of the photolysis laser focal volume. Supplementary Table 1 shows focal volume sizes and their associated errors. While the numerical model shows that the members of the H-atom pulse-train are already 100 times shorter than any previously produced, still shorter H-atom pulses are possible. Three factors influence H-atom pulse duration: the f/number of the optical system used to focus the photolysis laser, the means of producing the spatial distribution of photolysis frequencies and the choice of photolysis wavelength. Proper focusing of the photolysis pulse can further shorten the H-atom pulse. Referring to Fig. 1 , smaller f/numbers yield sharper foci for the individual frequency components of the beam; but the Rayleigh length of the focus also decreases. Hence, the size of the HI molecular beam must match the Rayleigh length; otherwise, H-atoms generated outside the focal region degrade the pulse duration. In other words, the narrower we choose the molecular beam width, the smaller the f/number can be and the shorter the H-atom pulse. In this work, we employed a rather large f-number (f/114) for the photolysis laser pulse. In an improved set-up, for example using f/13 optics, which matches a molecular beam width of 0.25 mm, the numerical model predicts a pulse-duration of 690 ps. Further shortening is possible with smaller f/number optics, but requires reducing the photolysis volume further along the laser propagation direction. In Supplementary Note 1 , we show that the spatial frequency distribution produced by the grating/lens combination— Supplementary Equation (19) —deviates from the ideal distribution, given by Supplementary Equation (15) . See also Supplementary Fig. 1 . We further show that a realizable adaptive optics set-up—shown in Supplementary Fig. 2 —can significantly improve the frequency distribution—see the Methods section and Supplementary Fig. 3 . Repeating the calculation of the previous paragraph assuming an ideal spatial frequency distribution, the numerical model predicts a further reduction of the H–atom pulse duration to 350 ps. Substantially shorter H-atom pulses are possible at shorter photolysis wavelengths, both due to the increased H-atom speeds and the fact that shorter wavelength light can be focused more tightly producing a better defined pulse. We note that bunch-compression photolysis scales favourably with increasing photon energy. In the limit where the photolysis photon energy, hv , is equal to the final translational energy of the H-atom, the pulse width scales as v −3/2 . Consider a bunch-compression experiment at λ =157.6 nm, where high-gain harmonic generation (HGHG) free electron lasers (FEL) [21] , [22] could be used and where HI photodissociation has been thoroughly studied [23] , [24] . We repeated the simulation above with an ideal spatial frequency distribution and f/17 optics. We reduced the collision area at the surface to 0.5 × 0.5 mm 2 , using a molecular beam width of 0.25 mm. The simulation predicts a 3.8 eV H-atom pulse with a 110 ps (FWHM) duration. We emphasize the advantage of the larger photolysis volume made possible by bunch-compression photolysis compared with simple focusing. Without bunch-compression, the size of the photolysis volume must be small, particularly in the direction of the H-atom propagation. With bunch-compression, we can achieve more than a 1000-fold increase in the size of the photolysis volume along the H-atom propagation direction without broadening the H-atom pulse. This allows more HI molecules to be used in the experiment and suppresses possible competitive multi-photon processes, such as multi-photon ionization. By tuning the photolysis wavelength to stronger HI absorptions, using higher photolysis pulse energies or by using other molecules with larger absorption cross-sections, H-atom beam intensities exceeding 4 × 10 16 H-atoms cm −2 s −1 can be achieved in a 110-ps pulse. See Supplementary Note 4 . With bunch-compression photolysis, it is now possible to produce ultra-short atomic pulses with sufficient intensity to be used in combination with synchronized light, ion, electron or molecular pulses. It is now possible to initiate collisions with unprecedented time precision and to probe atomic interactions with short-lived interaction partners. While this technique is not capable of directly following atomic scale motion as has become routine using fs-laser pulses, the ideas presented here show how to overcome the most challenging barrier to a new class of time-resolved dynamics experiments, opening new frontiers in the study of neutral matter. 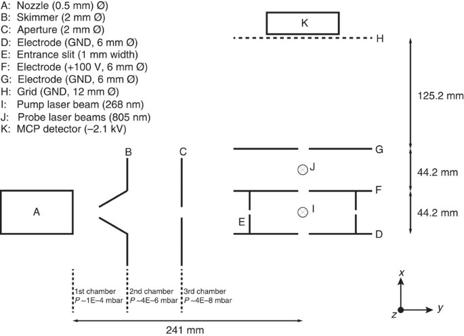Figure 4: Schematic drawing of the experimental set-up. The experiment is performed in a set of three differentially pumped vacuum chambers, which are connected by holes with 2 mm diameter and pumped by turbo molecular pumps (STP-301C, Edwards). In the first two chambers a collimated pulsed molecular beam of pure HI (stagnation pressure 2 bar, propagates alongy-axis) is generated using a water-cooled solenoid valve25with a 0.5 mm diameter opening (A) at a repetition rate of 50 Hz and a skimmer (Beam Dynamics, 2 mm diameter, (B) before it passes through a hole to the third chamber (C). This chamber contains the ion optics (D–H) each 1.5 mm thick (indicated distances refer to centres of each ion optic) with the micro channel plate detector (MCP, chevron set-up, Burle Industries, (K). The ion optics assembly consists of three electrodes with 6 mm apertures in the centre (D,F,G). A rectangular (1 × 10 mm) slit at (E), with its long dimension parallel to the H-atom flight direction(x-axis) and its short dimension along the laser propagation (z) axis, serves to narrow the dissociation volume along the photolysis laser propagation direction (z-axis). The HI beam is photodissociated at (I). Electrode (F) serves as a filter that only transmits neutral fragments. Hydrogen atoms reaching the bunch-compression point (J) are ionized with the probe laser (propagates alongz-axis). Between electrodes (F) and (G) the H+produced by the probe laser are accelerated into an approximately field-free drift region (G,H) before they enter the MCP detector. In the lower right corner, the coordinate system for the modelling is shown. Experimental Set-up Figure 4 shows a detailed schematic of the instrument used in this work. It consists of specialized laser systems and vacuum chambers. Figure 4: Schematic drawing of the experimental set-up. The experiment is performed in a set of three differentially pumped vacuum chambers, which are connected by holes with 2 mm diameter and pumped by turbo molecular pumps (STP-301C, Edwards). In the first two chambers a collimated pulsed molecular beam of pure HI (stagnation pressure 2 bar, propagates along y -axis) is generated using a water-cooled solenoid valve [25] with a 0.5 mm diameter opening (A) at a repetition rate of 50 Hz and a skimmer (Beam Dynamics, 2 mm diameter, (B) before it passes through a hole to the third chamber (C). This chamber contains the ion optics (D–H) each 1.5 mm thick (indicated distances refer to centres of each ion optic) with the micro channel plate detector (MCP, chevron set-up, Burle Industries, (K). The ion optics assembly consists of three electrodes with 6 mm apertures in the centre (D,F,G). A rectangular (1 × 10 mm) slit at (E), with its long dimension parallel to the H-atom flight direction (x -axis) and its short dimension along the laser propagation ( z ) axis, serves to narrow the dissociation volume along the photolysis laser propagation direction ( z -axis). The HI beam is photodissociated at (I). Electrode (F) serves as a filter that only transmits neutral fragments. Hydrogen atoms reaching the bunch-compression point (J) are ionized with the probe laser (propagates along z -axis). Between electrodes (F) and (G) the H + produced by the probe laser are accelerated into an approximately field-free drift region (G,H) before they enter the MCP detector. In the lower right corner, the coordinate system for the modelling is shown. Full size image Laser systems The fs-laser pulses used for bunch-compression photolysis and H-atom detection are produced by a Ti:sapphire oscillator (Vitesse, Coherent, 100-fs pulse width) amplified in two, synchronized 1-kHz regenerative Ti:sapphire amplifiers (RGA). The 80 MHz output of the oscillator serves as the clock for triggering the Pockels-cells of each RGA. In this way, the output of the probe RGA can be delayed by up to 900 μs in steps of 12.5 ns=(80 MHz) −1 with respect to the output of the photolysis RGA. An additional continuously tunable delay of 0–13.5 ns is achieved with a multi-pass optical delay stage. The RGA used for photolysis (Libra, Coherent) is frequency tripled producing 0.45 mJ per pulse at 268 nm. The second RGA is home-built and produces 1 mJ per pulse at 805 nm. To produce a spatial frequency distribution, the pump pulses are dispersed with a ruled 2,400 lines mm −1 grating (Spectrogon) optimized for a 50° angle of incidence and focused onto the molecular beam with an AR-coated fused silica lens (f=250 mm). Owing to the accompanying temporal broadening associated with the time delay imposed by the grating, the effective pulse duration of the laser light experienced by the HI molecules at the line focus is on the order of 10 ps. The energy reaching the photolysis volume was typically 40 μJ per pulse. The probe pulses are focused with a f=200 mm fused silica lens to the bunch-compression spot. Vacuum chambers and molecular beam system A detailed schematic diagram of the experimental set-up used in this work is shown in Fig. 4 . The experiment is realized in a set of three vacuum chambers each pumped by a turbo-molecular pump. In the first chamber, a pulsed HI molecular beam (duration ~200 μs) of pure HI (stagnation pressure 2 bar) is generated using a water cooled solenoid valve with a 0.5 mm diameter opening at a repetition rate of 50 Hz. It is then collimated by a 2-mm electro-formed skimmer (Beam Dynamics), differentially pumped in the second chamber and passes through a 2-mm aperture to the third chamber, where the bunch-compression photolysis and H-atom pulse detection are carried out. The bunch-compression photolysis laser pulse crosses the HI molecular beam 24 cm from the nozzle in the third chamber and a tightly focused probe laser pulse ionizes the H-atoms 44.57 mm away by a sixth order non-resonant process. A micro-channel plate (MCP) is used to detect the ions. The ion optics assembly consists of three electrodes, which are used to prevent any charged particles produced by the photolysis laser from reaching the MCP. Furthermore, ions produced by the probe laser are detected such that their arrival time at the MCP is both mass and velocity sensitive. Thus, we can easily discriminate our desired H-atom photolysis signal, which results from H-atoms travelling with 10.89 km s −1 , from ions of other mass as well as H + produced from background gas. The MCP signal was acquired by an averaging oscilloscope (DPO 3034, Tektronix) and transferred to a PC. The optical delay between the pump and probe pulses was scanned to obtain the time profile of the H-atom pulse produced in the experiment. For each pump-probe delay, the desired H + signal arising from HI photolysis was integrated over 512 molecular beam pulses. Background was measured by delaying the molecular beam pulse by 500 μs with respect to the laser pulses. Supplementary Table 1 gives additional experimental conditions. Numerical model The numerical model and the theory behind it are described in Supplementary Note 2 . How to cite this article: Kaufmann, S. et al . Generation of ultra-short hydrogen atom pulses by bunch-compression photolysis. Nat. Commun. 5:5373 doi: 10.1038/ncomms6373 (2014).